CD91-dependent programming of T-helper cell responses following heat shock protein immunization The immunogenic heat shock proteins (HSPs) gp96, hsp70 and calreticulin (CRT) bind to CD91 on antigen-presenting cells (APCs) for cross-presentation of the HSP-chaperoned peptides. This event leads to priming of T-cell responses. Here we show that CD91 serves as a signalling receptor for these HSPs, allowing for the maturation of APCs, secretion of cytokines and priming of T-helper (Th) cells. Specifically, CD91 is phosphorylated in response to HSPs in a unique pattern and phospho-CD91 triggers signalling cascades to activate nuclear factor-kappa B. Each HSP–CD91 interaction on APCs stimulates a unique cytokine profile, which dictates priming of specific Th cell subsets. Thus, in a transforming growth factor-β tumour microenvironment, immunization with CRT, but not gp96 or hsp70, primes Th17-cell responses in a CD91-dependent manner. These results are important for development of T-cell responses in situ in tumour-bearing hosts and for vaccination against cancer and infectious disease. Heat shock proteins (HSPs) gp96, hsp70, hsp90 and calreticulin (CRT) prime immune responses that have been utilized for immunotherapy of cancer and infectious disease [1] , [2] , [3] . These immune responses, which are primarily T-cell responses primed against the peptides that these HSPs chaperone [4] , [5] , mediate their effects through cytotoxicity of antigen-expressing cells. In several antigenic systems tested in vitro and in vivo , dendritic cells and macrophages acquire extracellular HSPs via the receptor CD91 and cross-present the peptides that are naturally chaperoned by these HSPs on major histocompatibility complex molecules [6] , [7] , [8] , [9] , [10] , [11] , [12] , providing signal 1 for T-cell priming. Less is known about how HSPs stimulate APCs to provide costimulation. APCs stimulated with HSPs have been shown to activate nuclear factor-kappa B (NF-κB), release proinflammatory cytokines and upregulate the expression of CD40, B7 and major histocompatibility complex II, the classic markers of dendritic cell maturation [13] . Although CD91 is the key receptor for HSP-mediated endocytosis and cross-presentation of chaperoned peptides, the HSP receptor that is responsible for these innate responses in APCs is not known. Several candidates have been proposed. The reports that Toll-like receptor (TLR)2/4 are HSP receptors [14] , [15] have been controversial, as the results have been indistinguishable from endotoxin-mediated responses. Complete removal of contaminating endotoxin from HSP preparations, the use of good laboratory practice-grade HSP, or the use of TLR2/4 −/− cells or mice have shown no dependence on TLRs [16] . In addition, affinity chromatography and crosslinking experiments have not shown any association of HSPs with TLRs [6] . As CD91 was the primary receptor isolated in those studies we have asked the question whether CD91 is involved in innate responses elicited by HSPs thereby functioning as a signalling receptor. We show, first, CD91 is the receptor for the HSP-induced innate responses. Specifically we show that activation of NF-κB in APCs by gp96, hsp70 and CRT is dependent on CD91 and the phosphorylation of its cytosolic domain. Interestingly although all the three HSPs engage CD91 on APCs, gp96 and CRT utilize different phosphorylation sites on the receptor from hsp70 for the activation of NF-κB. Second, the unique cytokine profile resulting from each HSP–CD91 interaction determines the nature of the effector T cells that are ultimately primed. In a transforming growth factor-beta (TGF-β)-secreting tumour microenvironment, CRT, but not gp96 or hsp70, immunization is able to prime T-helper (Th)17 cells in draining lymph nodes. We show that interleukin (IL)-6 and tumour necrosis factor (TNF)-α, but not IL-21 or IL-23 (ref. 17 ), are necessary for CRT-mediated Th17 priming. The results show how each immunogenic HSP can direct different T-cell responses through a single receptor CD91, and are important in understanding the initiation of immune responses when HSPs are released into the extracellular environment from tumour or infected cells [13] , [18] . These data also directly impact clinical trials in which HSPs are used for cancer immunotherapy [19] , [20] . Thus, CD91 functions as a signalling receptor for the immunogenic HSPs and the resulting immune responses can be skewed to various Th subsets. HSP-mediated NF-κB activation is CD91 dependent Immunogenic HSPs, gp96, hsp70 and CRT bind to CD91 (refs 6 , 7 ). To determine whether CD91 was a signalling receptor for HSPs, gp96, hsp70 and CRT were purified from mouse tissues in an endotoxin-free procedure to apparent homogeneity as characterized by SDS–PAGE ( Fig. 1a ) and immunoblotting ( Fig. 1b ). RAW264.7 cells, which express high levels of CD91 ( Fig. 1c ), were transfected with the NF-κB reporter construct such that NF-κB activation could be monitored by a luciferase assay. Reporter-transfected RAW264.7 cells were pulsed with increasing doses of gp96, hsp70 or CRT as indicated for 30 mins. NF-κB activation was measured in the supernatants and plotted as fold increase over PBS-pulsed cells. All three HSPs activated NF-κB in a dose-dependent manner ( Fig. 1d ). In a time course experiment, gp96, hsp70 and CRT activated NF-κB rapidly and achieved maximum response within 60 mins and waned thereafter ( Fig. 1e ). The kinetics of NF-κB activation by lipopolysaccharide (LPS) was different; 1 EU of LPS did not elicit a response at 60 mins but rather achieved its maximum response at 6 h, fully consistent with previous observations [13] . To determine whether activation of NF-κB was dependent on CD91, transfected RAW264.7 cells were incubated with HSPs in the presence or absence of anti-CD91 antibody or control IgG. Before use in this experiment the amount of anti-CD91 antibody was carefully titrated and optimized ( Fig. 1f ). A dose of 20 μg (per 100 μl reaction volume) was considered the maximal blocking concentration that did not compromise cell viability. We found that anti-CD91 antibody was able to fully abrogate NF-κB activation (to background levels set by antibody alone groups) when cells were pulsed with gp96 or CRT ( Fig. 1g ; Student's t -test, P <0.001, P <0.002, respectively). The NF-κB signal was partially abrogated ( ∼ 50%) when cells were pulsed with hsp70 (Student's t -test, P <0.01; Fig. 1g ). Neither antibody by itself activated NF-κB. These data demonstrate that CD91 was functioning as a signalling receptor for the immunogenic HSPs and that this activation was not due to undetectable amounts of endotoxin. 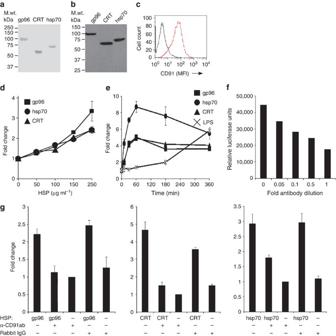Figure 1: HSP-mediated NF-κB activation is CD91 dependent. (a) Gp96, calreticulin (CRT) or hsp70 was purified and 1 μg was analysed on a 10% SDS–PAGE. (b) Gp96, CRT or hsp70 was immunoblotted with their corresponding antibodies. (c) The macrophage cell line RAW264.7 was stained with rabbit anti-CD91 IgG (red) or control rabbit IgG (black) and then with a fluorescein isothiocyanate-labelled secondary antibody. Mean fluorescent intensities (MFIs) are measured. (d) RAW264.7 cells transfected with NF-κB–luciferase reporter were pulsed with gp96, CRT or hsp70 at different concentrations and luminescence was measured after 30 min. Results are plotted as fold change in luciferase activity of HSP-pulsed cells over that of PBS-pulsed cells. (e) RAW264.7 cells transfected with NF-κB–luciferase reporter were pulsed with equimolar amounts of gp96, CRT or hsp70, 1 EU LPS or PBS for different times and luminescence was measured. Results are plotted as fold change in luciferase activity of HSP-pulsed or LPS-pulsed cells over that of PBS-pulsed cells. (f) RAW264.7 cells transfected with the NF-κB–luciferase reporter were incubated with 100 μg ml−1of gp96 without (0) anti-CD91 antibody or with increasing antibody concentrations. NF-κB activation was plotted as relative luciferase units. (g) RAW264.7 cells transfected with the NF-κB–luciferase reporter plasmid were pulsed with gp96, CRT or hsp70 in the presence or absence of the anti-CD91 IgG or control rabbit IgG. Control cells were incubated with the antibodies alone without HSPs. The relative luciferase units were measured after 30 min incubation and plotted as fold change over anti-CD91 antibody alone. Error bars in (d–g) represent the s.d. of triplicates. Figure shows one of at least three independent experiments with similar results. Figure 1: HSP-mediated NF-κB activation is CD91 dependent. ( a ) Gp96, calreticulin (CRT) or hsp70 was purified and 1 μg was analysed on a 10% SDS–PAGE. ( b ) Gp96, CRT or hsp70 was immunoblotted with their corresponding antibodies. ( c ) The macrophage cell line RAW264.7 was stained with rabbit anti-CD91 IgG (red) or control rabbit IgG (black) and then with a fluorescein isothiocyanate-labelled secondary antibody. Mean fluorescent intensities (MFIs) are measured. ( d ) RAW264.7 cells transfected with NF-κB–luciferase reporter were pulsed with gp96, CRT or hsp70 at different concentrations and luminescence was measured after 30 min. Results are plotted as fold change in luciferase activity of HSP-pulsed cells over that of PBS-pulsed cells. ( e ) RAW264.7 cells transfected with NF-κB–luciferase reporter were pulsed with equimolar amounts of gp96, CRT or hsp70, 1 EU LPS or PBS for different times and luminescence was measured. Results are plotted as fold change in luciferase activity of HSP-pulsed or LPS-pulsed cells over that of PBS-pulsed cells. ( f ) RAW264.7 cells transfected with the NF-κB–luciferase reporter were incubated with 100 μg ml −1 of gp96 without (0) anti-CD91 antibody or with increasing antibody concentrations. NF-κB activation was plotted as relative luciferase units. ( g ) RAW264.7 cells transfected with the NF-κB–luciferase reporter plasmid were pulsed with gp96, CRT or hsp70 in the presence or absence of the anti-CD91 IgG or control rabbit IgG. Control cells were incubated with the antibodies alone without HSPs. The relative luciferase units were measured after 30 min incubation and plotted as fold change over anti-CD91 antibody alone. Error bars in ( d–g ) represent the s.d. of triplicates. Figure shows one of at least three independent experiments with similar results. Full size image HSPs use alternative tyrosine phosphorylation sites on CD91 Signalling receptors typically utilize tyrosine phosphorylation to transmit signals intracellularly. CD91 consists of an extracellular α-chain non-covalently associated with a β-chain. The β-chain harbours the transmembrane and intracellular domains with two tyrosine phosphorylation (NPXY) motifs [21] . To test for phosphorylation of CD91, RAW264.7 cells were pulsed with gp96, hsp70 or CRT and the β-chain was immunoprecipitated. The β-chain immunoprecipitates were probed via immunoblotting with anti-phosphotyrosine (pTyr) antibodies ( Fig. 2a ). We found that with each HSP, the β-chain was phosphorylated, whereas PBS-pulsed cells did not show such phosphorylation. Equal amounts of β-chain were immunoprecipitated in each group. 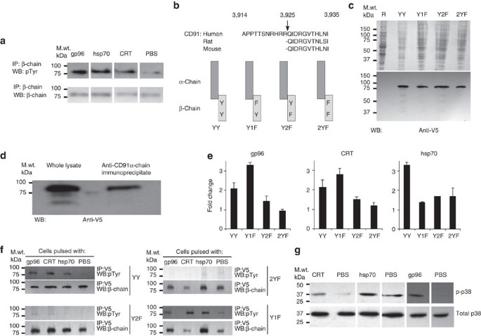Figure 2: HSPs use alternative tyrosine phosphorylation sites on CD91. (a) RAW264.7 cells were pulsed with gp96, CRT, hsp70 or PBS for 30 min and CD91 was immunoprecipitated with mouse anti-CD91 β-chain antibody. Immunoprecipitates were probed with 4G10/PY20 anti-phosphotyrosine antibodies (pTyr) or with β-chain-specific antibody (β-chain). (b) Alignment of the CD91 sequence from human, rat and mouse showing the highly conserved furin cleavage site, which forms the α- and β-chains. The two NPXY motifs in the β-chain of CD91, where the tyrosines can be phosphorylated for intracellular signalling, is shown. Mutations of these tyrosines individually (YIF, Y2F) or together (2YF) to phenylalanine along with wild-type (YY) construct were cloned in fusion with the V5 epitope. Constructs are depicted. (c) The four constructs were transfected separately in RAW264.7 carrying the NF-κB–luciferase reporter. The cell lysates of the untransfected (R) or transfected cells were analysed by SDS–PAGE and immunoblotted with anti-V5 antibody to probe for the expression of the 85-kDa exogenous β-chain. (d) The α-chain of CD91 was immunoprecipitated from the cell lysate of RAW264.7 cells transfected with the representative YY construct using anti-CD91 α-chain antibody. The cell lysate and the immunoprecipitate were analysed by SDS–PAGE and immunoblotted with anti-V5. Similar results were obtained with the other constructs. (e) Each of the doubly transfected RAW264.7 cells (NF-κB–luciferase reporter and β-chain mutant) was pulsed with gp96, CRT, hsp70 or PBS. The relative luciferase units were measured after 30 min incubation and plotted as fold change in luciferase activity of HSP-pulsed cells over that of PBS-pulsed cells. Error bars represent s.d. of triplicates. (f) RAW264.7 transfected with wild-type β-chain (YY) or with β-chain mutants (Y2F, 2YF or YIF) was pulsed with gp96, CRT or hsp70 or PBS for 30 min. The β-chains were immunoprecipitated from cell lysates with anti-V5 antibody and probed for pTyr or β-chain. (g) RAW264.7 was pulsed with gp96, CRT, hsp70 or PBS for 30 min and cell lysates obtained. The lysates were immunoblotted with anti-phospho-p38 (p-p38) and anti-p38 (total p38) antibodies. Data are representative of at least three independent experiments with similar results. Figure 2: HSPs use alternative tyrosine phosphorylation sites on CD91. ( a ) RAW264.7 cells were pulsed with gp96, CRT, hsp70 or PBS for 30 min and CD91 was immunoprecipitated with mouse anti-CD91 β-chain antibody. Immunoprecipitates were probed with 4G10/PY20 anti-phosphotyrosine antibodies (pTyr) or with β-chain-specific antibody (β-chain). ( b ) Alignment of the CD91 sequence from human, rat and mouse showing the highly conserved furin cleavage site, which forms the α- and β-chains. The two NPXY motifs in the β-chain of CD91, where the tyrosines can be phosphorylated for intracellular signalling, is shown. Mutations of these tyrosines individually (YIF, Y2F) or together (2YF) to phenylalanine along with wild-type (YY) construct were cloned in fusion with the V5 epitope. Constructs are depicted. ( c ) The four constructs were transfected separately in RAW264.7 carrying the NF-κB–luciferase reporter. The cell lysates of the untransfected (R) or transfected cells were analysed by SDS–PAGE and immunoblotted with anti-V5 antibody to probe for the expression of the 85-kDa exogenous β-chain. ( d ) The α-chain of CD91 was immunoprecipitated from the cell lysate of RAW264.7 cells transfected with the representative YY construct using anti-CD91 α-chain antibody. The cell lysate and the immunoprecipitate were analysed by SDS–PAGE and immunoblotted with anti-V5. Similar results were obtained with the other constructs. ( e ) Each of the doubly transfected RAW264.7 cells (NF-κB–luciferase reporter and β-chain mutant) was pulsed with gp96, CRT, hsp70 or PBS. The relative luciferase units were measured after 30 min incubation and plotted as fold change in luciferase activity of HSP-pulsed cells over that of PBS-pulsed cells. Error bars represent s.d. of triplicates. ( f ) RAW264.7 transfected with wild-type β-chain (YY) or with β-chain mutants (Y2F, 2YF or YIF) was pulsed with gp96, CRT or hsp70 or PBS for 30 min. The β-chains were immunoprecipitated from cell lysates with anti-V5 antibody and probed for pTyr or β-chain. ( g ) RAW264.7 was pulsed with gp96, CRT, hsp70 or PBS for 30 min and cell lysates obtained. The lysates were immunoblotted with anti-phospho-p38 (p-p38) and anti-p38 (total p38) antibodies. Data are representative of at least three independent experiments with similar results. Full size image To determine which tyrosine in the two NPXY motifs of the β-chain of CD91 was utilized for signal transduction we took advantage of the inherent processing of CD91 to mutate the tyrosines. The 600-kDa polypeptide chain of CD91 is cleaved in the endoplasmic reticulum at a furin cleavage site (conserved in rodents and humans) into the α- and β-chains, which then re-associate non-covalently ( Fig. 2b ) [22] , [23] . We cloned the β-chain (YY), attached the endoplasmic reticulum signal sequence of the α-chain and a C-terminal V5 epitope by PCR to this construct and used site-directed mutagenesis to change the membrane proximal (Y1F) or the distal (Y2F) or both (2YF) tyrosine(s) in the NPXY motifs to phenylalanine as depicted ( Fig. 2b ). The constructs were expressed in RAW264.7 cells, which endogenously express wild-type α- and β-chains. Similar levels of expression were observed for each construct in immunoblotting of RAW264.7 cell lysates for the V5-epitope tag ( Fig. 2c ). We tested whether the mutant β-chain constructs associated with the endogenous α-chain. The endogenous α-chain was immunoprecipitated from cells expressing each of the various mutants and the immunoprecipitates were probed with anti-V5-epitope antibody. A representative immunoblot in Figure 2d shows that the expressed β-chain (YY) coimmunoprecipitated with the endogenous α-chain. We tested the dependence of the HSP on each tyrosine for signal transduction. RAW264.7 cells doubly transfected with the NF-κB reporter construct and one of the respective mutant CD91 β-chain was pulsed with gp96, hsp70 or CRT or PBS. We found that gp96 and CRT both required the membrane distal but not the proximal tyrosine for NF-κB activation because activation was significantly abrogated in Y2F cells ( Fig. 2e ). NF-κB was slightly enhanced in Y1F cells. On the other hand, hsp70 required both the proximal and distal tyrosines for NF-κB activation because activation was abrogated in both Y2F and Y1F cells ( Fig. 2e ). No further significant reduction in NF-κB activation was observed when (2YF) cells with both tyrosines mutated were pulsed with any HSP. These results show that although gp96, hsp70 and CRT all signal through CD91, they function so in different ways by utilizing either the membrane distal (gp96, hsp70, CRT) or the proximal (hsp70) NPXY motifs. We confirmed the results in Figure 2e by immunoprecipitations of the β-chain and immunoblotting for pTyr. The loss of NF-κB signal in cells transfected with Y2F and 2YF after pulsing with each HSPs observed in Figure 2e is also seen by immunoblotting where there is a decrease in phosphorylation signal with tyrosine mutations ( Fig. 2f ). In addition to activation of NF-κB we examined HSP-pulsed RAW264.7 cells for activation of other signalling molecules. We observed that phospho-p38 MAPK was increased in cells pulsed with gp96, hsp70 or CRT when compared with PBS-pulsed cells ( Fig. 2g ). Total p38 in all groups remained the same. No specific phosphorylation of Akt, ERK1/2, JNK1/2/3, MKK3/6 or MAK2 was observed. HSP–CD91 interactions provide distinct cytokine profiles The differences observed in the way the HSPs use the receptor CD91 suggested that the outcomes of the signalling cascades initiated by receptor phosphorylation would be different for each HSP. We analysed an array of cytokines and chemokines secreted, first, by the RAW264.7 cell line in a cytokine array profiler ( Table 1 ). RAW264.7 cells were pulsed with gp96, hsp70 or CRT. Supernatants were collected after 20 h and analysed by immunoblot arrays. Two observations were made: first, cytokines released included known NF-κB-dependent (for example, IL-6, IL-1β) and -independent genes (for example, granulocyte colony-stimulating factor), and second, the cytokines released in response to each HSP were distinct (for example, CXCL11) and overlapping (for example, IL-1β, IL-12p70). These results suggest that multiple and NF-κB independent pathways exist for APC activation and that the differences seen at the CD91 phosphorylation level are translated to the respective cytokine profiles. Next, we analysed five cytokines, known to be important for Th cell differentiation and/or proliferation, by the more quantitative method of enzyme-linked immunosorbent assay (ELISA). We used inherent (unmanipulated) murine APCs to mimic what would happen in vivo in response to extracellular HSPs. Peritoneal exudate cells (PECs), which as a population express high levels of CD91 ( Fig. 3a ) and cross-present HSP-chaperoned peptides [7] , [24] , were isolated from naïve mice and immediately pulsed with equimolar amounts of gp96, hsp70, CRT or PBS. Supernatants were collected after 20 h and analysed by ELISA for IL-1, IL-6, IL-21, IL-23 and TNF-α ( Fig. 3b–d ). The incubations were performed in the presence or absence of anti-CD91 antibody. Several observations were made: first, IL-1β was released in comparable amounts by PECs pulsed with gp96, CRT or hsp70 ( Fig. 3b ); second, gp96- or CRT-pulsed PECs released IL-6, whereas hsp70-pulsed PECs released significantly less IL-6 ( Fig. 3c ); third, CRT-pulsed PECs released five times more TNF-α than PECs pulsed with gp96 or hsp70 ( Fig. 3d ); and fourth, all three cytokines released by PECs in response to HSPs were CD91-dependent, as anti-CD91 antibody significantly inhibited these responses ( Fig. 3b–d ; Student's t -test, P <0.05 comparing with and without anti-CD91 antibody in all groups). No IL-21 or IL-23 was detected when PECs were pulsed with any of the HSPs. In a second set of experiments we tested the dependence of cytokine secretion on NF-κB activation. PECs were isolated from naïve mice and immediately pulsed with gp96, hsp70, CRT, LPS or PBS in the presence or absence of the NF-κB inhibitor Cardamonin. Supernatants were collected after 20 h and analysed by ELISA for IL-1β, IL-6 and TNF-α ( Fig. 3e–g ). In each situation where HSP- or LPS-pulsed PECs released the cytokines IL-1β, IL-6 or TNF-α, Cardamonin was able to significantly abrogate the response (Student's t -test, P <0.05 comparing with and without Cardamonin in all groups). Cytokines released by HSP-pulsed PECs were therefore CD91- and NF-κB-dependent. Table 1 Distinct cytokine release profiles by HSPs. 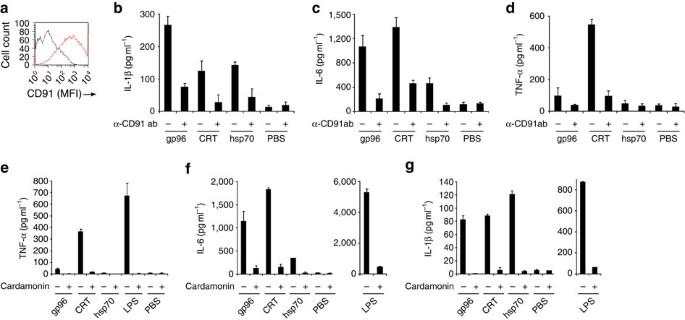Figure 3: HSP-CD91 interactions provide distinct cytokine profiles. (a) Peritoneal exudate cells obtained from C57BL/6 mice were stained with rabbit anti-CD91 antibody (red) or control IgG (black) and then with the fluorescein isothiocyanate-labelled secondary antibody. PECs obtained from C57BL/6 mice were incubated for 20 h with gp96, CRT or hsp70 or PBS. Incubations were carried out in the presence (+) or absence (−) of anti-CD91 antibody. Supernatants were collected and assayed by ELISA for (b) IL-1β, (c) IL-6 or (d) TNF-α. PECs obtained from C57BL/6 mice were incubated for 20 h with gp96, CRT or hsp70 or 1 EU LPS or PBS. Incubations were carried out in the presence (+) or absence (−) of 10 μM of the NF-κB inhibitor Cardamonin. Supernatants were collected and assayed by ELISA for (e) TNF-α, (f) IL-6 or (g) IL-1β. Error bars inb–grepresent s.d. of triplicates. Figure represents one of at least twoaor threeb–gindependent experiments with similar results. Full size table Figure 3: HSP-CD91 interactions provide distinct cytokine profiles. ( a ) Peritoneal exudate cells obtained from C57BL/6 mice were stained with rabbit anti-CD91 antibody (red) or control IgG (black) and then with the fluorescein isothiocyanate-labelled secondary antibody. PECs obtained from C57BL/6 mice were incubated for 20 h with gp96, CRT or hsp70 or PBS. Incubations were carried out in the presence (+) or absence (−) of anti-CD91 antibody. Supernatants were collected and assayed by ELISA for ( b ) IL-1β, ( c ) IL-6 or ( d ) TNF-α. PECs obtained from C57BL/6 mice were incubated for 20 h with gp96, CRT or hsp70 or 1 EU LPS or PBS. Incubations were carried out in the presence (+) or absence (−) of 10 μM of the NF-κB inhibitor Cardamonin. Supernatants were collected and assayed by ELISA for ( e ) TNF-α, ( f ) IL-6 or ( g ) IL-1β. Error bars in b–g represent s.d. of triplicates. Figure represents one of at least two a or three b–g independent experiments with similar results. Full size image Calreticulin primes Th17 cells in a TGF-β microenvironment HSP immunization typically targets lymph nodes distant from the tumour, where the release of proinflammatory cytokines such as IL-1β, TNF-α and IL-12 by targeted APCs skew responses to the Th1/CTL phenotype [1] , [3] , [4] , [13] . However, targeting HSP immunization to local APCs and tumour-draining lymph nodes with different cytokine milieus may generate alternate phenotypes. We asked the question whether HSP immunization at draining lymph nodes, could bias responses to a Th17 phenotype in a TGF-β microenvironment [25] , given the robust IL-6 production from gp96 or CRT-treated PECs ( Fig. 3c ). The EL.4 tumour expresses TGF-β [26] , and was used as a constant source of TGF-β in vivo . We confirmed TGF-β expression by our EL.4 cell line by flow cytometry ( Fig. 4a ), consistent with previous studies [26] . In addition, TGF-β expression was confirmed by real-time and RT–PCR, alongside the housekeeping gene hypoxanthine-guanine phosphoribosyl transferase (HPRT). 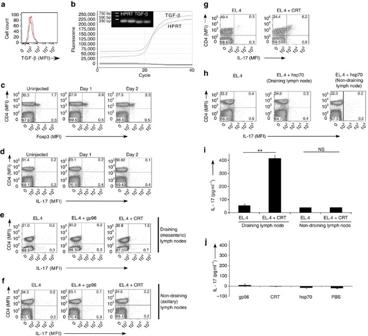Figure 4: Calreticulin primes Th17 cells in a TGF-β microenvironment. (a) EL.4 cells were analysed by flow cytometry for intracellular TGF-β (red). Black line is irrelevant isotype antibody. (b) Expression level of TGF-β1 in EL.4 cells was analysed by real-time RT-PCR and compared with the positive control hypoxanthine-guanine phosphoribosyl transferase. Agarose gel electrophoresis of RT-PCR for hypoxanthine-guanine phosphoribosyl transferase (214 bp) and TGF-β1 (145 bp) is shown in duplicates. (c) C57BL/6 mice were injected intraperitoneally with EL.4 cells on day 0 and the mesenteric lymph nodes were collected from groups of mice on every day and stained for CD4 and Foxp3. (d) Mice were administered EL.4 cells on day 0 and the mesenteric lymph nodes analysed by flow cytometry for IL-17. (e) Mice were administered EL.4 cells alone or with gp96 or CRT. The mesenteric lymph nodes were collected on day 6 and analysed by flow cytometry for IL-17. (f) Mice were administered EL.4 cells alone or with gp96 or CRT. The non-draining lymph nodes were collected on day 6 and analysed by flow cytometry for IL-17. (g) C57BL/6 mice were administered EL.4 cells alone or with CRT. The mesenteric lymph nodes were collected on day 6 and stimulated for 4 h with phorbol myristate acetate and ionomycin. Cells were analysed by flow cytometry for IL-17. (h) Mice were administered EL.4 cells alone or with hsp70. The draining or non-draining (axillary) lymph nodes were collected on day 6 and analysed by flow cytometry for IL-17. (i) Mesenteric or axillary lymph node CD4+cells were culturedex vivofor 3 days with anti-CD3 and irradiated spleen and supernatants were tested for IL-17A by ELISA. Error bars represent s.d. of triplicates (Student'st-test **P<0.01; NS, nonsignificant). (j) Mice were administered HSPs or PBS. The mesenteric lymph nodes were collected on day 6 and were culturedex vivofor 3 days with anti-CD3 and irradiated spleen. Culture supernatants were tested for IL-17A. Error bars represent s.d. of triplicates. Figure is representative of one set of a total of four (c,d), or eight (e–h) or three sets of mice (i,j), tested in independent experiments. Figure 4b shows that TGF-β is expressed by real-time PCR and by electrophoresis of RT–PCR. To determine whether these levels of TGF-β had any immune relevance we injected the EL.4 tumour into the peritoneum of mice. Mesenteric lymph nodes were collected from mice every 24 h after injection and proliferation of CD4 + Foxp3 + cells was monitored. We found that this population increased over the course of 2 days ( Fig. 4c ) (in four mice per group tested; Student's t -test, P =0.018). No difference in the Th17 population was observed as a result of tumour inoculation over this period (in four mice per group tested; Student's t -test, P =0.39; Fig. 4d ). Mice were then immunized with EL.4 tumour cells alone or simultaneously with gp96 or CRT. Draining mesenteric ( Fig. 4e ) or non-draining axillary ( Fig. 4f ) lymph nodes were collected after 6 days and stained for Th17 cells. Coimmunization of EL.4 and CRT primed Th17 cells in draining lymph nodes (in six of eight responders; Student's t -test, P =0.047), whereas coimmunization of EL.4 tumour with gp96 did not prime Th17 cells (in eight mice tested, Student's t -test, P =0.216; Fig. 4e ). No Th17 responses were observed in non-draining lymph nodes ( Fig. 4f ). The Th17 cells observed in EL.4+CRT-immunized mice could be significantly expanded ex vivo by stimulation with phorbol myristate acetate/ionomycin for 4 h (with Golgi plug) to reveal a distinct CD4 + IL17 + population (in eight mice tested, Student's t -test, P <0.002; Fig. 4g ). No such phenotype was observed in mice immunized with EL.4 cells alone. Mice coimmunized with EL.4 tumour and hsp70 did not prime Th17 cells in draining (in eight mice tested, Student's t -test, P =0.28) or non-draining lymph nodes ( Fig. 4h ). To confirm the presence of a population of Th17 cells in the EL.4+CRT-immunized mice, draining or non-draining lymph node cells were collected, sorted for CD4 + cells and stimulated ex vivo with plate-bound anti-CD3 and irradiated spleen for 3 days. Culture supernatants were collected and tested for IL-17A by ELISA. Culture supernatants from this group were observed to have eightfold higher amounts of IL-17A compared with lymph node cells derived from mice immunized with EL.4 cells alone ( Fig. 4i ). In addition, no IL-17A was detected in non-draining lymph nodes (Student's t -test, P >0.1). For other controls, mice were immunized with HSPs alone, that is, in the absence of TGF-β (no EL.4 cells). No Th17 cells were detected (Student's t -test, P >0.2 any HSP compared with PBS; Fig. 4j ). Figure 4: Calreticulin primes Th17 cells in a TGF-β microenvironment. ( a ) EL.4 cells were analysed by flow cytometry for intracellular TGF-β (red). Black line is irrelevant isotype antibody. ( b ) Expression level of TGF-β1 in EL.4 cells was analysed by real-time RT-PCR and compared with the positive control hypoxanthine-guanine phosphoribosyl transferase. Agarose gel electrophoresis of RT-PCR for hypoxanthine-guanine phosphoribosyl transferase (214 bp) and TGF-β1 (145 bp) is shown in duplicates. ( c ) C57BL/6 mice were injected intraperitoneally with EL.4 cells on day 0 and the mesenteric lymph nodes were collected from groups of mice on every day and stained for CD4 and Foxp3. ( d ) Mice were administered EL.4 cells on day 0 and the mesenteric lymph nodes analysed by flow cytometry for IL-17. ( e ) Mice were administered EL.4 cells alone or with gp96 or CRT. The mesenteric lymph nodes were collected on day 6 and analysed by flow cytometry for IL-17. ( f ) Mice were administered EL.4 cells alone or with gp96 or CRT. The non-draining lymph nodes were collected on day 6 and analysed by flow cytometry for IL-17. ( g ) C57BL/6 mice were administered EL.4 cells alone or with CRT. The mesenteric lymph nodes were collected on day 6 and stimulated for 4 h with phorbol myristate acetate and ionomycin. Cells were analysed by flow cytometry for IL-17. ( h ) Mice were administered EL.4 cells alone or with hsp70. The draining or non-draining (axillary) lymph nodes were collected on day 6 and analysed by flow cytometry for IL-17. ( i ) Mesenteric or axillary lymph node CD4 + cells were cultured ex vivo for 3 days with anti-CD3 and irradiated spleen and supernatants were tested for IL-17A by ELISA. Error bars represent s.d. of triplicates (Student's t -test ** P <0.01; NS, nonsignificant). ( j ) Mice were administered HSPs or PBS. The mesenteric lymph nodes were collected on day 6 and were cultured ex vivo for 3 days with anti-CD3 and irradiated spleen. Culture supernatants were tested for IL-17A. Error bars represent s.d. of triplicates. Figure is representative of one set of a total of four ( c,d ), or eight ( e–h ) or three sets of mice ( i,j ), tested in independent experiments. Full size image Th17 priming is dependent on CD91 and IL-6 and TNF-α We have demonstrated the requirement of CD91 for HSP signalling in APCs in vitro ( Figs 1g , 2 and 3 ). We tested whether CD91 signalling was required for Th17 priming in vivo by administering CD91-targeting small interfering RNA (siRNA) to mice intraperitoneally. PECs were collected every 24 h and CD91 expression was monitored by flow cytometry. We observed that CD91 expression was diminished by 30 and 73% on day 1 and day 2 post administration, respectively ( Fig. 5a ). Cells began to recover CD91 expression after day 2. We then designed an experimental scheme to test the dependence of Th17 priming on CD91 ( Fig. 5b ). CD91-targeting siRNA was administered intraperitoneally on day −2 and day 0 to ensure CD91 expression remained diminished spanning CRT introduction. EL.4 with or without CRT was then administered on day 0. Draining (mesenteric) lymph nodes were collected on day 6, sorted for CD4 + cells, cultured with plate-bound anti-CD3 and irradiated spleen cells and tested for IL-17A on day 9. The high IL-17A levels observed with EL.4+CRT was effectively abrogated when CD91-targeting siRNA was administered ( Fig. 5c ). Administration of EL.4 with or without siRNA was set as the background IL-17A level. These data were confirmed by flow cytometry on day 6. Draining lymph node cells from EL.4+CRT-immunized mice demonstrated a significant population of Th17 cells, which was diminished in the presence of CD91-siRNA (in nine pairs of mice tested in three independent experiments, Student's t -test, P <0.04; Fig. 5d ). No Th17 responses were detected in mice administered with EL.4 with or without siRNA. The cytokines that were tested in Figure 3 , were those that have been shown to be necessary for or supported Th17 differentiation and/or proliferation [27] , [28] . We therefore tested the role of IL-6 and TNF-α in CRT-mediated Th17 priming. IL-6-deficient or wild-type mice were immunized with EL.4 alone or coimmunized with EL.4+CRT. Priming of Th17 cells observed in wild-type mice was abrogated in IL-6-deficient mice (three mice per group in three independent experiments, Student's t -test, P =0.48; Fig. 5e ), indicating that IL-6 was necessary for the CRT-mediated Th17 priming. We tested the role of TNF-α in two independent assays ( Fig. 5f ). First, mice were administered EL.4 and CRT in the presence or absence of anti-TNF-α antibody. Further antibody was administered on day 2. Draining (mesenteric) lymph nodes were collected on day 6, sorted for CD4 + cells, cultured with plate-bound anti-CD3 and irradiated spleen cells and tested for IL-17A on day 9. The robust IL-17A production observed in the EL.4+CRT group of mice was effectively abrogated by anti-TNF-α antibody ( Fig. 5g ). Second, mice were administered EL.4 and gp96 together with recombinant TNF-α. Further rTNF-α was given on day 2. Draining (mesenteric) lymph nodes were collected on day 6, sorted for CD4 + cells, cultured with plate-bound anti-CD3 and irradiated spleen cells and tested for IL-17A on day 9. In the presence of rTNF-α, gp96 was able to prime cells to produce IL-17A ( Fig. 5h ). Our results show that Th17 priming by CRT was dependent on CD91, IL-6 and TNF-α. 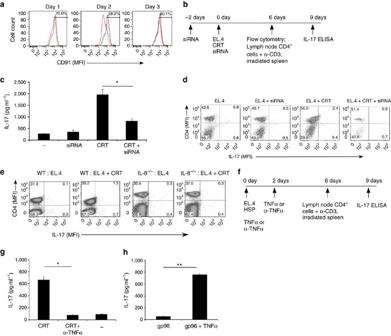Figure 5: Th17 priming is dependent on CD91 and IL-6 and TNF-α. (a) Mice were inoculated intraperitoneally with CD91-targeting siRNA for various times. PECs were analysed by flow cytometry every 24 h. (b) Experimental scheme for determining the dependence of Th17 priming on CD91. CD91-targeting siRNA was administered to mice before (day −2) and during EL.4+CRT administration (day 0). (c) Draining lymph nodes were collected on day 6. CD4+cells were isolated and stimulated with α-CD3 and irradiated spleenex vivo. Culture supernatants were tested on day 9. Controls include mice administered EL.4 alone (−) and EL.4+siRNA (siRNA). Error bars represent s.d. of triplicates (Student'st-test *P<0.05). (d) Draining lymph node cells from mice administered EL.4+CRT, with or without siRNA, were collected on day 6 and stained for CD4 and IL-17 and analysed by flow cytometry. Controls include mice administered EL.4 alone and EL.4+siRNA. (e) Wild-type or IL-6-deficient mice were inoculated with EL.4 alone or EL.4+CRT. Draining lymph node cells from all mice were collected on day 6 and analysed by flow cytometry. Figure is representative of one pair of a total of three pairs of mice. (f) Experimental scheme for determining the dependence of Th17 priming on TNF-α. Mice were administered EL.4 cells together with gp96 or CRT. Mice receiving EL.4 and CRT were administered α-TNF-α antibody on day 0 and day 2. Mice receiving EL.4 and gp96 were administered rTNF-α on day 0 and day 2. CD4+cells were isolated from the lymph node cells on day 6 and stimulated with α-CD3 and irradiated spleenex vivo. Culture supernatants were tested on day 9 for IL-17A. (g) ELISA for IL-17A from mice administered EL4+CRT and α-TNF-α antibody. Controls include mice administered only EL.4+CRT (CRT) or EL.4 alone (−) (Student'st-test *P<0.003). (h) ELISA for IL-17A from mice administered EL4+gp96 and rTNF-α. Mice were administered EL.4 and gp96 (gp96) as a control (Student'st-test **P<0.004). Figure represents one of three independent experiments with similar results inc,gandh. Figure 5: Th17 priming is dependent on CD91 and IL-6 and TNF-α. ( a ) Mice were inoculated intraperitoneally with CD91-targeting siRNA for various times. PECs were analysed by flow cytometry every 24 h. ( b ) Experimental scheme for determining the dependence of Th17 priming on CD91. CD91-targeting siRNA was administered to mice before (day −2) and during EL.4+CRT administration (day 0). ( c ) Draining lymph nodes were collected on day 6. CD4 + cells were isolated and stimulated with α-CD3 and irradiated spleen ex vivo . Culture supernatants were tested on day 9. Controls include mice administered EL.4 alone (−) and EL.4+siRNA (siRNA). Error bars represent s.d. of triplicates (Student's t -test * P <0.05). ( d ) Draining lymph node cells from mice administered EL.4+CRT, with or without siRNA, were collected on day 6 and stained for CD4 and IL-17 and analysed by flow cytometry. Controls include mice administered EL.4 alone and EL.4+siRNA. ( e ) Wild-type or IL-6-deficient mice were inoculated with EL.4 alone or EL.4+CRT. Draining lymph node cells from all mice were collected on day 6 and analysed by flow cytometry. Figure is representative of one pair of a total of three pairs of mice. ( f ) Experimental scheme for determining the dependence of Th17 priming on TNF-α. Mice were administered EL.4 cells together with gp96 or CRT. Mice receiving EL.4 and CRT were administered α-TNF-α antibody on day 0 and day 2. Mice receiving EL.4 and gp96 were administered rTNF-α on day 0 and day 2. CD4 + cells were isolated from the lymph node cells on day 6 and stimulated with α-CD3 and irradiated spleen ex vivo . Culture supernatants were tested on day 9 for IL-17A. ( g ) ELISA for IL-17A from mice administered EL4+CRT and α-TNF-α antibody. Controls include mice administered only EL.4+CRT (CRT) or EL.4 alone (−) (Student's t -test * P <0.003). ( h ) ELISA for IL-17A from mice administered EL4+gp96 and rTNF-α. Mice were administered EL.4 and gp96 (gp96) as a control (Student's t -test ** P <0.004). Figure represents one of three independent experiments with similar results in c , g and h . Full size image Immunization with HSPs elicits potent Th1/CTL anti-tumour immune response HSPs engage CD91 on APCs that allows for cross-priming of the chaperoned peptide antigen [6] , [7] . These events have been well characterized. One question that has remained unresolved was the mechanism by which HSPs provided signal 2, necessary for priming T cells and what alternative T-cell responses may be obtained. We describe here that the receptor CD91 has a central role in signal transduction by HSPs via activation of p38 MAPK and NF-κB. HSPs utilize different phosphorylation sites on CD91, which may account for distinct cytokine profiles released by APCs in response to respective HSPs. These cytokine patterns (for CRT) are shown to be capable of directing T-cell responses to a Th17 phenotype. CD91 was shown to be the endocytic receptor for the immunogenic HSPs including gp96, hsp90, hsp70 and CRT, and it is required for cross-presentation of HSP-chaperoned peptides and tumour immunity [6] , [7] , [8] , [9] , [10] , [11] , [12] . In one study in which CD91 independence of HSP responses was described [29] , the results were shown to be a result of several lacunae in experimental design [8] . Once these lacunae are addressed, CD91 is shown to have a vital role in the interaction of gp96 with APCs. CD91 is a typical scavenger receptor, which binds and internalizes multiple structurally and functionally diverse ligands. It is synthesized as a 600-kDa type I transmembrane protein, which, during transit to the cell surface, is processed by furin [22] into a 515-kDa α- and a 85-kDa β-subunit in the trans-Golgi network [23] . A number of CD91 ligands, including tPA, α 2 M, apoE, MMP-9 and connective tissue growth factor, have recently been shown to activate signalling cascades after binding to CD91 (refs 30 , 31 , 32 , 33 , 34 , 35 ). For example, the activation of both MAPK and NF-κB has been observed following binding of α 2 M to CD91, which in turn induces MMP-9 production [35] . In these studies, CD91 may regulate the cellular microenvironment by its ability to endocytose diverse extracellular mediators, facilitating endocytosis of other transmembrane receptors involved in cell signalling or directly regulating cell signalling and gene transcription via adaptor proteins. Given the emerging role of CD91 in signalling, our data extends the role of CD91 to immune system regulation through its interaction with extracellular HSPs. Basu et al ., [13] described the activation and nuclear translocation of NF-κB in response to HSPs. We now show that the activation happens through CD91. By selective mutations of the two tyrosines of CD91, gp96 and CRT were determined to utilize membrane-proximal tyrosine 4508, while hsp70 utilizes both tyrosine 4474 and tyrosine 4508 to transduce signals. Unlike LDLR, the NPXY motifs of CD91 do not have a role in endocytosis [36] but are rather involved in binding pTyr-binding domains of intracellular signalling proteins [37] , [38] , [39] , [40] . We are yet to confirm adaptor proteins, but a number of candidates exist in the literature; PI3K, Shp-2, CSK, Shc-3, Grb-2 have been shown to associate with tyrosine 4508 of CD91 in response to various (non-HSP) ligands [41] . These candidates may be used by the HSPs to transmit signals. For hsp70, there may be other binding partners that interact with tyrosine 4474. Downstream, we show that p38 MAPK is activated. Others kinases, ERK and PI3K, are also phosphorylated in a CD91-dependent manner [42] . These signalling proteins along with NF-κB activation and p38 phosphorylation may constitute a single or multiple pathways. The full signalling cascade is currently under investigation. We have been extremely careful in these studies with respect to endotoxin contamination. TLR2/4 have been suggested to be involved in HSP-mediated signalling and activation of APCs. However, a large body of literature, including our data presented here suggests that the TLRs have no contribution to HSP-mediated signalling events (for review see Binder [16] ). The current literature on HSP signalling presents a disjointed picture due to the use of APCs manipulated in vivo or in vitro [13] , cell lines and HSPs with varying levels of endotoxin contamination [14] , [15] . We have used the macrophage cell line to examine the influence of the signalling cascade on cytokine secretion and unmodified PECs from naïve mice to investigate what the cytokine milieu would be if (endotoxin free) HSPs were present in the extracellular space in the peritoneum. Both NF-κB-dependent and -independent cytokine genes were observed to be activated, suggesting that more than a single signalling pathway was being utilized. IL-12, TNF-α and IL-1β are transcribed from genes that are regulated by NF-κB [43] , [44] , [45] , [46] and direct immune responses to the Th1/CTL phenotype. We observed that the proinflammatory cytokine IL-6 was released by PECs in response to gp96 or CRT but to a much lesser degree by hsp70. The difference between gp96 or CRT and hsp70 could stem from the difference noted at the receptor tyrosine phosphorylation level, although a direct connection between the two events has not yet been made. Indeed IL-6 expression can be regulated by p38 MAPK alone [47] or in combination with NF-κB-dependent events [48] . This may suggest that an additional NF-κB independent signalling cascade may be invoked by CRT and/or gp96. In support of this, CRT, but to a much lesser degree gp96 or hsp70, stimulated PECs to release TNF-α. There seems to be a reciprocal development pathway for Treg and Th17 cells with IL-6 having a pivotal role by inhibiting the generation of Treg cells and inducing the production of Th17 cells. In a TGF-β tumour microenvironment, IL-6 secreted in response to CRT was necessary to direct priming of Th17 cells as demonstrated by the lack of such priming in IL-6 −/− mice. However, IL-6 was insufficient by itself because gp96, which stimulates PECs to release similar amounts of IL-6, did not prime Th17 cells. However, TNF-α production in response to CRT correlated with the ability to prime Th17. Hsp70 did not prime Th17 cells probably due to the lack of IL-6 and TNF-α production. IL-21 or IL-23 can function as a polarizing cytokine for Th17 priming in the absence of IL-6 or can enhance the effects of IL-6 (ref. 17 ). Both IL-21 and IL-23 were not released by PECs in response to any HSP. The priming of Th17 cells by CRT is currently being tested in various autoimmune disease models but it might also have a role in anti-tumour immunity [49] . Extracellular HSPs, introduced via vaccination or released from cells, thus, have the ability to prime T-cell responses of the Th1 (refs 3 , 18 , 50 ), Th2 (ref. 51 ), Treg [52] , [53] or Th17 type ( Fig. 6 ). The resulting phenotype will depend on the relative abundance of each HSP in the extracellular environment, affinity of each HSP for CD91, the APC type and the contributions of other cell types in the microenvironment. These results have far reaching implications from long-term non-progressor HIV patients [50] , cancer immunotherapy [19] , [20] and initiation of immune responses to tumours [13] , [18] . 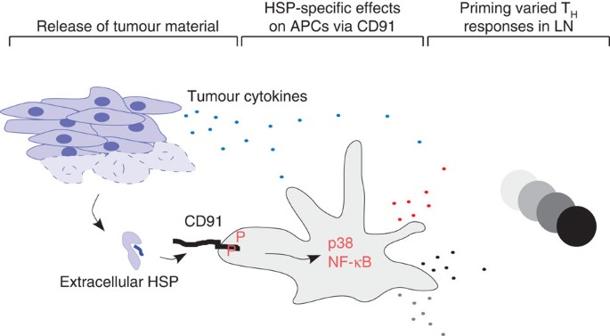Figure 6: A model of Th cell priming by extracellular HSPs. The release of HSPs from tumour cells (or introduced through vaccination) into the extracellular environment has the potential to stimulate APCs through CD91. The APCs will advertise HSP-specific effects through a unique pattern of costimulation (cytokines described here and costimulatory molecules13) in the draining lymph nodes where they prime Th cell subsets of different types. These effects are nevertheless influenced by other cytokines the tumour cells themselves may release such as TGF-β. Figure 6: A model of Th cell priming by extracellular HSPs. The release of HSPs from tumour cells (or introduced through vaccination) into the extracellular environment has the potential to stimulate APCs through CD91. The APCs will advertise HSP-specific effects through a unique pattern of costimulation (cytokines described here and costimulatory molecules [13] ) in the draining lymph nodes where they prime Th cell subsets of different types. These effects are nevertheless influenced by other cytokines the tumour cells themselves may release such as TGF-β. Full size image Molecular biology methods Total RNA was isolated from mouse liver by using RNeasy Mini Kit (Qiagen) and treated with RNase-free DNase to eliminate any potential genomic DNA contamination. Aliquots of 1 μg of total RNA were used for first-strand cDNA synthesis by using the Omniscript RT kit (Qiagen). The cDNA was used for amplification (in the 5′–3′ direction) by the primer pair CCCCTGCTCAGTGCTCTAGTTGCTGCTCAGATCGACCGCGGAGTCACCCACCTCAATATTTC (CD91NT1) and CGCCAAGGGATCTCCTATCTCGTCTTCAGGTCCCCG (CD91CT), and the resulting PCR product was used for amplification by the primer pair CCGATGCTGACCCCGCCGTTGCTGCTGCTGCTGCCCCTGCTCAGTGCTCTGGTTGCTGCTCAG (CD91NT2) and CD91CT for mouse CD91 β-chain. CD91NT1 and CD91NT2 primers add the nucleotides encoding the signal sequence of the CD91 α-chain, which ensures the expression of the exogenous β-chain in the same compartment as the α-chain. PCR amplification was performed by using 2× Mango Mix (Bioline USA Inc.) for 30 cycles (94 °C for 30 s, 55 °C for 30 s and 72 °C for 75 s). After amplification, the 1.8-kb PCR product was cloned into pEF6/V5-His-TOPO vector (Invitrogen) containing a V5 epitope at the carboxyl terminal and transformed into Escherichia coli. The wild-type CD91 protein has two tyrosine residues at 4474 (NPTY) and 4508 (NPVY) so the wild-type β-chain construct was used to make the tyrosine to phenylalanine mutants of CD91 β-chain by using the QuikChange XL Site-Directed Mutagenesis Kit (Stratagene). The individual mutation of the membrane proximal- and distal-tyrosine was termed as Y1F and Y2F, respectively. The wild-type and the mutant with both tyrosine mutated to phenyalanine was termed as YY and 2YF, respectively. RAW264.7 macrophages were stably transfected with each of the aforementioned plasmids by using Fugene6 transfection reagent (Roche Molecular Biochemicals). DNA sequencing was performed at Genewiz. Real-time PCR Total RNA was prepared from EL.4 cells using the RNeasy mini kit (Qiagen) according to the manufacturer's instruction. To avoid contamination with genomic DNA, RNA samples were treated with RNase-free DNAse I (Roche Diagnostics GmbH). To generate cDNA from cell culture samples, 500 ng of total RNA was reverse transcribed using iScript cDNA synthesis kit (Bio-Rad). cDNA was analysed by real-time PCR by using StepOne Real Time PCR system (Amersham). For amplification, QuantiTect TGF beta1 primers (Qiagen) or custom-synthesized hypoxanthine-guanine phosphoribosyl transferase primers (5′-GTAATGATCAGTCAACGGGGGAC-3′ forward; 5′-CCAGCAAGCTTGCAACCTTAACCA-3′ reverse) were used with the iQ SYBR Green supermix (Bio-Rad). For standard RT–PCR using the same primers, the following conditions were used: 35 cycles of 94 °C for 30 s, 55 °C for 30 s and 72 °C for 30 s. The PCR products were analysed by agarose gel electrophoresis in 1×TAE buffer (Bio-Rad). Cell culture RAW264.7 and 11H4 cells (American Type Culture Collection) were cultured in complete Dulbecco's modified Eagle's medium (1% sodium pyruvate, 1% penicillin and streptomycin, 1% glutamine, 1% non-essential amino acids, 0.1% 2-mercaptoethanol) and 10% fetal bovine serum (GIBCO/Invitrogen). The mouse lymphoma cell line EL.4 (ATCC) cells and PECs were cultured in complete RPMI with 5% fetal bovine serum. RAW264.7 cells transfected with the NF-κB–luciferase vector (pNFκB-MetLuc2) or β-chain mutants were grown in 0.4 g l −1 geneticin and 2 mg l −1 blasticidin, respectively. All cell cultures were maintained at 37 °C in a humidified atmosphere containing 5% CO 2 . To measure IL-17A levels, CD4 + T cells were purified from single suspensions of lymph node cells by negative selection (Miltenyi Biotec). CD4 + T cells were plated at equal numbers in anti-CD3 coated plates with irradiated spleen as a source of CD28 ligands in 24 well plates. Culture supernatants were collected on day 3 and used for IL-17A ELISA. For investigating the role of TNF-α, C57BL/6 mice were immunized at day 0 with a single intraperitoneal injection of 2×10 6 EL.4 cells with the following: 100 μg of gp96 or equimolar amounts of CRT, 100 μg of gp96 and 10 ng of rTNF-α (ThermoFisher) or equimolar amounts of CRT and 125 μg of anti-TNF-α antibody (Thermofisher). At day 2, another dose of rTNF-α and anti-TNF-α antibody was administered to the respective mice and the mice were killed at day 6. The mesenteric lymph nodes were collected and cell suspensions were used for IL-17A ELISA. Immunoprecipitation and immunoblotting Cells (1×10 6 ) were grown in P6 culture dishes and pulsed with the HSPs for 30 min. The cells were rinsed with cold PBS and lysed in 1 ml of NP40 Tris lysis buffer. Lysates were cleared by centrifugation at 10,000 g for 15 min in a microcentrifuge, incubated with 5 μl of polyclonal antiserum or 1 μg of monoclonal antibody for 1 h on ice and subsequently for 1 h with 100 μl of 10% protein G-Sepharose at 4 °C on an agitator. Sepharose beads were collected by centrifugation and washed four times with NP40 lysis buffer. Immunoprecipitates were boiled for 3 min in sodium dodecyl sulfate sample buffer and resolved by SDS–PAGE. Membranes were blocked for 1 h in Tris buffer with Tween and 5% dried milk, incubated with 1:1,000 dilution of polyclonal antisera in Tris buffer with Tween and 5% milk for 1 h followed by incubation with horseradish peroxidase-conjugated polyclonal IgG antibody (Sigma), all at room temperature. Reactive proteins were visualized by ECL (Amersham Pharmacia Biotech). The protein size was confirmed by molecular weight standards (Bio-Rad). Full-length immunoblots representing those in Figure 2 are shown in Supplementary Figure S1 . Purification of HSPs Calreticulin, hsp70 and gp96 were simultaneously purified from C57BL/6 mouse liver tissue according to previously described methods [1] , [2] , [3] . No recombinant HSPs were used in any experiment and all proteins had undetectable amounts of endotoxin present. Pulsing experiments in vitro were performed with 100 μg ml −1 of gp96 and equimolar amounts of CRT or hsp70 ( Figs 1 , 2 , 3 ). The amounts of HSPs used to pulse cells in vitro was estimated based on calculation of the average amount of HSP produced per cell (2–3 pg) and the average volume of a cell (50 μm). Mice were injected with 100 μg of gp96 or equimolar amounts of CRT or hsp70 ( Figs. 4 and 5 ) Expression of CD91 and knockdown using siRNA CD91 expression on RAW264.7 cells and PECs was measured by staining the cells with 5 μg of anti-CD91 antibody for 15 min on ice and after two washes with PBS, incubated with anti-rabbit-fluorescein isothiocyanate antibody. The cells were washed twice with PBS and analysed by flow cytometry. The CD91-targeting siRNA was obtained from Sigma; five sequences targeting various portions of the mRNA were mixed (1 nM each). To verify knockdown of CD91 in vivo , the siRNA was administered intraperitoneally and PECs were collected on days 1, 2 and 3 after injection. The cells were stained as mentioned above for CD91 expression, which showed highest decrease at day 2 after injection. To determine the dependence of Th17 priming on CD91, mice were injected with siRNA 2 days before and during injection of EL.4 or EL.4 and HSP. Mice and reagents Female C57BL/6 and B6.129S6-Il6tmKopf (IL6 −/− ) mice were obtained from Jackson Laboratory and housed in the DLAR at the University of Pittsburgh and were used under the IACUC guidelines after approval of the relevant protocols at the University of Pittsburgh. The following kits were obtained and used according to the manufacturer's recommendation: Ready to glow secreted luciferase reporter system (Clontech), Mouse Th17/Treg Phenotyping kit (BD Biosciences), Oligotex mRNA purification kit (Qiagen), Mouse cytokine array panel A and Human Phospho-MAPK array kit. Oligonucleotides were obtained from Eurofins MWG/Operon. The following antibodies were used: mouse anti-phospho-p38 MAPK (The180/Tyr182) (28B10), rabbit anti-p38 MAP Kinase antibody (Cell Signaling Technology), mouse anti-V5-HRP (Invitrogen), mouse anti-pTyr antibody clone 4G10 and clone PY20 (Millipore), anti-CD91 β-chain clone IgG-11H4 (ATCC), anti-TGF-β1, -β2, -β3-allophycocyanin (R&D Systems), Ready-set-Go mouse IL-21, IL-1β, IL-6, TNF-α, IL-23, IL-17A (homodimer) ELISA kits were from eBiosciences. Anti-CD3 antibody was a kind gift of Dr Michael Turner (University of Pittsburgh). Cardamonin was obtained from TOCRIS Biosciences and used at a concentration of 10 μM. CD91 blocking The anti-CD91 antibody was obtained from Agenus Inc., and was made by immunization of rabbits with the 95-amino acid N-terminal fragment of the α-chain of CD91. The IgG was purified from total serum of the immunized rabbit using the Melon gel IgG purification kit (Pierce). Unimmunized rabbit IgG was used as control antibody. Flow cytometry Mice were immunized with a single intraperitoneal injection of 2×10 6 EL.4 cells with or without 100 μg of gp96 or equimolar amounts of CRT or hsp70. The mice were killed 6 days after the injection and the peritoneum draining (mesenteric) or non-draining (axillary) lymph node were collected. Single-cell suspensions of the lymph node were stained for Th17/Treg phenotypes as recommended by the manufacturer (BD Pharmingen). In some experiments, cells were stimulated with phorbol myristate acetate (50 ng ml −1 ), ionomycin (1 μg ml −1 ) and Golgi plug for 4 h before staining. Samples were run on LSRII Flow Cytometer (BD Biosciences) and data were analysed by the FlowJo software. Statistical analysis P -values were obtained by Student's t -test. How to cite this article: Pawaria, S. & Binder, R.J. CD91-dependent programming of T-helper cell responses following heat shock protein immunization. Nat. Commun. 2:521 doi: 10.1038/ncomms1524 (2011).